Scaffold function of long non-coding RNAHOTAIRin protein ubiquitination Although mammalian long non-coding (lnc)RNAs are best known for modulating transcription, their post-transcriptional influence on mRNA splicing, stability and translation is emerging. Here we report a post-translational function for the lncRNA HOTAIR as an inducer of ubiquitin-mediated proteolysis. HOTAIR associates with E3 ubiquitin ligases bearing RNA-binding domains, Dzip3 and Mex3b, as well as with their respective ubiquitination substrates, Ataxin-1 and Snurportin-1. In this manner, HOTAIR facilitates the ubiquitination of Ataxin-1 by Dzip3 and Snurportin-1 by Mex3b in cells and in vitro , and accelerates their degradation. HOTAIR levels are highly upregulated in senescent cells, causing rapid decay of targets Ataxin-1 and Snurportin-1, and preventing premature senescence. These results uncover a role for a lncRNA, HOTAIR , as a platform for protein ubiquitination. Eukaryotic gene expression is tightly regulated by post-transcriptional mechanisms controlled by non-coding RNAs (ncRNAs) and by RNA-binding proteins (RBPs). Among the small ncRNAs, microRNAs (miRNAs) typically repress gene expression by inhibiting the translation or promoting the decay of target mRNAs [1] . miRNA-mediated silencing is elicited by components of the RNA-induced silencing complex such as argonaute 2 (Ago2), which cleaves target mRNAs, remodels mRNA-containing ribonucleoprotein complexes and affects mRNA translation and stability [2] , [3] . Long ncRNAs (lncRNAs) have been implicated primarily in transcriptional regulation by modulating the activity of transcription factors and by serving as scaffolds for assembling transcriptional regulators [4] . A number of post-transcriptional functions for lncRNAs are also emerging, with examples of lncRNAs titrating miRNAs and RBPs, guiding ribonucleoprotein (RNP) complexes, sequestering splicing factors, modulating mRNA decay and suppressing target mRNA translation [5] , [6] , [7] , [8] , [9] . One of the best-studied RBPs is human antigen R (HuR), a ubiquitous protein that stabilizes and modulates the translation of many target mRNAs. In a recent study, Mukherjee et al. [10] used Photoactivatable-Ribonucleoside-Enhanced Crosslinking and Immunoprecipitation (PAR-CLIP) sequencing to identify a variety of additional HuR target transcripts, including pre-mRNAs, lncRNAs and miRNAs. Among the non-coding ligands of HuR was let7 (lethal-7), a miRNA first described in nematodes and highly conserved among species; in mammalian cells, let7 regulates many processes, including cell proliferation, development, tumorigenesis and apoptosis [11] . The discovery of HuR-associated small ncRNAs and lncRNAs prompted us to investigate these interactions in detail, as well as to study the regulation and consequences of these complexes. Here, we report that HuR associates with the lncRNA HOTAIR (HOX antisense intergenic RNA) and lowers its stability by recruiting the let7-Ago2 complex. We show evidence that HOTAIR forms complexes with two E3 ubiquitin ligases bearing RNA-binding domains, Dzip3 and Mex3b, and HOTAIR also interacts with their respective ubiquitination substrates, Ataxin-1 and Snurportin-1. By facilitating the formation of these complexes, HOTAIR promotes the ubiquitination of Ataxin-1 by Dzip3 and Snurportin-1 by Mex3b and increases their degradation. When HuR levels decline in cellular processes such as cell senescence, HOTAIR is stable and displays a previously unrecognized post-translational function as a modulator of ubiquitin-mediated proteolysis. HuR enhances the interaction of Ago2 with let7 Using fluorescence anisotropy-based binding assays, we investigated the binding of purified recombinant HuR with fluorescein-tagged let7b and let7i, two of the HuR-bound miRNAs identified by PAR-CLIP analysis. HuR formed direct complexes with let7 substrates consistent with single-site binding models, with K d =1.6 nM for let7b and K d =9.6 nM for let7i ( Fig. 1a,b ). HuR binding to let7b was particularly strong, comparable to the affinity measured for a similarly sized AU-rich element, a hallmark substrate for HuR [12] , whereas binding to let7i was weaker. We also studied the interaction of endogenous HuR with miRNA in HeLa (human cervical carcinoma) cells by RNP immunoprecipitation (RIP) analysis, which identifies HuR-bound transcripts by employing an anti-HuR antibody and mild immunoprecipitation (IP) conditions that preserve HuR-RNA complexes. In HeLa cell lysates, HuR RIP and northern blot analysis revealed that mature let7 miRNA was enriched in HuR IP samples but not in control IgG IP samples, further indicating that HuR was capable of interacting with endogenous mature let7 present in cytoplasmic lysate, whereas a negative control RNA ( U6 ) was not ( Fig. 1c ). 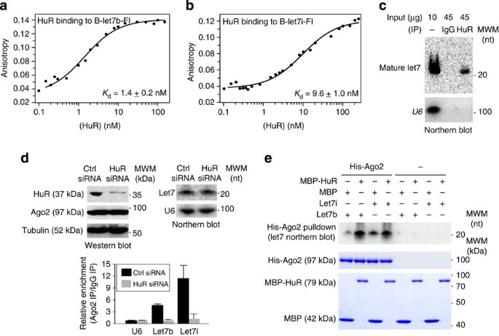Figure 1:HuR and let7/Ago2 cooperatively bindHOTAIR. (a,b)In vitrobinding of untagged recombinant HuR to fluorescein-tagged let7b and let7i was analysed by fluorescence anisotropy. RNP complex affinity was resolved using a single-site binding model (solid lines). (c) HuR interaction with endogenous mature let7 in HeLa cell lysates was assessed by RIP using anti-HuR and IgG antibodies, RNA isolation and northern blot analysis; the abundant RNAU6was assessed as negative control. (d) Forty-eight hours after transfecting HeLa cells with the siRNAs shown, protein levels, total levels of let7 and loading controlU6, and let7b-Ago2 and let7i-Ago2 associations were assessed by WB, northern blot and RIP analyses, respectively. Graph represents the means and s.d. from three independent experiments. (e) Pulldown analysis using recombinant His-tagged Ago2, let7b or let7i and MBP or MBP-HuR. Let7b and let7i abundance was assessed by northern blot analysis; proteins in the reaction were visualized using Coomassie blue stain. Figure 1: HuR and let7/Ago2 cooperatively bind HOTAIR . ( a , b ) In vitro binding of untagged recombinant HuR to fluorescein-tagged let7b and let7i was analysed by fluorescence anisotropy. RNP complex affinity was resolved using a single-site binding model (solid lines). ( c ) HuR interaction with endogenous mature let7 in HeLa cell lysates was assessed by RIP using anti-HuR and IgG antibodies, RNA isolation and northern blot analysis; the abundant RNA U6 was assessed as negative control. ( d ) Forty-eight hours after transfecting HeLa cells with the siRNAs shown, protein levels, total levels of let7 and loading control U6 , and let7b-Ago2 and let7i-Ago2 associations were assessed by WB, northern blot and RIP analyses, respectively. Graph represents the means and s.d. from three independent experiments. ( e ) Pulldown analysis using recombinant His-tagged Ago2, let7b or let7i and MBP or MBP-HuR. Let7b and let7i abundance was assessed by northern blot analysis; proteins in the reaction were visualized using Coomassie blue stain. Full size image The strong binding of HuR and let7 suggested that HuR might functionally affect the association between Ago2 and let7, perhaps enhancing or inhibiting Ago-let7 interactions. To test these possibilities, we silenced HuR in HeLa cells using specific small interfering (si)RNA and measured let7b and let7i bound to Ago2 by RIP analysis followed by reverse transcription (RT) and real-time, quantitative (q)PCR analysis of small RNAs. Our results indicated that Ago2 binding to let7b and let7i was reduced (whereas Ago2 levels were not) when HuR was silenced, suggesting that HuR facilitated Ago2-let7 interactions ( Fig. 1d ). In vitro binding assays supported this hypothesis, as Ago2 (His-Ago2) interactions with let7b and let7i were enhanced in the presence of HuR (MBP-HuR; Fig. 1e ). These results suggest that HuR binds let7 and increases Ago2–let7 complexes. HuR interacts with HOTAIR and promotes its decay PAR-CLIP identified many lncRNAs as HuR target transcripts [10] . Among them, lincRNA-p21 was rendered unstable through its interaction with HuR, an effect dependent on the recruitment of let7 to lincRNA-p21 (ref. 9 ). A RIP-based screen to identify other lncRNAs associated with HuR revealed that HOTAIR was highly enriched (~18-fold) in HuR IP compared with IgG IP, as measured by RT-qPCR analysis of the RNA present in the IP material (normalized to the levels of GAPDH mRNA, encoding a housekeeping protein) ( Fig. 2a , Supplementary Fig. S1a ). By contrast, there was no enrichment in IP samples using an antibody against the RBP AUF1 ( Fig. 2a ); additional RBPs screened are in Supplementary Fig. S1b,c . A full-length (FL) biotinylated HOTAIR transcript was synthesized using a plasmid construct [13] and tested for binding to HuR in vitro . Pulldown with streptavidin-coated beads followed by Coomassie staining showed that recombinant Maltose-Binding Protein (MBP)-HuR, but not MBP alone, associated with the HOTAIR(FL) biotinylated RNA; a control biotinylated RNA ( GAPDH 3′ UTR ) did not associate with MBP-HuR ( Fig. 2b ). To map the site of interaction of HuR with HOTAIR , HeLa cell lysates were subjected to limited digestion with RNase T1 (Methods), so that G residues protected by an RBP would remain preferentially uncleaved. Following HuR IP, the fragments associated with HuR and protected from degradation were identified by RT and qPCR analysis using 23 primer pairs ( Supplementary Table S1 ) that scanned the HOTAIR transcript in overlapping ~150 nucleotide-long segments ( Fig. 2c ). As shown in Fig. 2d , HuR binding was greatest at segments 11 and 12, spanning nucleotides ~1,028–1,272, as confirmed by crosslinking IP (CLIP) analysis ( Supplementary Fig. S2a,b ) and by in vitro binding assays ( Supplementary Fig. S2f ). Minor binding was also seen for 5′ segments 3 and 4 (~223–471) and for several 3′ segments ( Fig. 2d ). 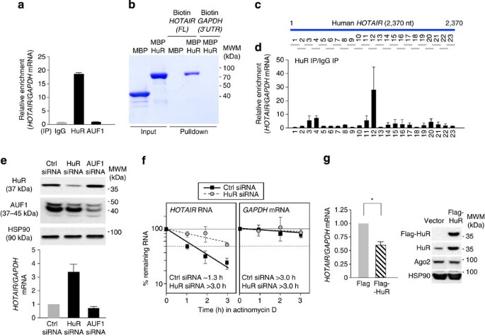Figure 2:HuR and let7/Ago2 promoteHOTAIRdecay. (a) RIP analysis of HeLa cell lysates to measure the interaction of HuR and AUF1 withHOTAIRandGAPDHmRNA (encoding a housekeeping protein), were quantified using RT-qPCR and represented as enrichment in RBP IP compared with IgG IP. (b) A biotinylated fragment spanning the FL ofHOTAIRwas used for pulldown analysis after incubation with MBP or MBP-HuR and was detected by staining with Coomassie blue; the interaction of MBP-HuR with a negative control transcript (biotinylatedGAPDH3′UTR) was included. (c,d) Schematic (c) ofHOTAIRand the segments assayed (grey lines) after RNase T1 digestion; HuR IP followed by RT-qPCR amplification was used to identify RNA segments associated with HuR (d). (e,f) Forty-eight hours after transfecting HeLa cells with the siRNAs indicated, the levels of HuR, AUF1 and loading control HSP90 were assessed by WB analysis, the steady-state levels ofHOTAIRandGAPDHmRNA by RT-qPCR (e), and the half-lives (t1/2) ofHOTAIRandGAPDHmRNA were quantified by measuring the rate of decline in transcript levels after adding actinomycin D (f). (g) Forty-eight hours after overexpressing HuR in HeLa cells,HOTAIRlevels were measured by RT-qPCR and normalized toGAPDHmRNA levels. Ina,e–g, the graphs represent the means and s.d. from three independent experiments; (d) the graph is representative from three experiments; data are the means and s.d. *P<0.05 using Student’st-test. Figure 2: HuR and let7/Ago2 promote HOTAIR decay. ( a ) RIP analysis of HeLa cell lysates to measure the interaction of HuR and AUF1 with HOTAIR and GAPDH mRNA (encoding a housekeeping protein), were quantified using RT-qPCR and represented as enrichment in RBP IP compared with IgG IP. ( b ) A biotinylated fragment spanning the FL of HOTAIR was used for pulldown analysis after incubation with MBP or MBP-HuR and was detected by staining with Coomassie blue; the interaction of MBP-HuR with a negative control transcript (biotinylated GAPDH 3′UTR) was included. ( c , d ) Schematic ( c ) of HOTAIR and the segments assayed (grey lines) after RNase T1 digestion; HuR IP followed by RT-qPCR amplification was used to identify RNA segments associated with HuR ( d ). ( e , f ) Forty-eight hours after transfecting HeLa cells with the siRNAs indicated, the levels of HuR, AUF1 and loading control HSP90 were assessed by WB analysis, the steady-state levels of HOTAIR and GAPDH mRNA by RT-qPCR ( e ), and the half-lives ( t 1/2 ) of HOTAIR and GAPDH mRNA were quantified by measuring the rate of decline in transcript levels after adding actinomycin D ( f ). ( g ) Forty-eight hours after overexpressing HuR in HeLa cells, HOTAIR levels were measured by RT-qPCR and normalized to GAPDH mRNA levels. In a , e – g , the graphs represent the means and s.d. from three independent experiments; ( d ) the graph is representative from three experiments; data are the means and s.d. * P <0.05 using Student’s t -test. Full size image To study the influence of HuR on HOTAIR expression, we silenced HuR or AUF1 in HeLa cells ( Fig. 2e , Supplementary Fig. S3 ). Compared with HOTAIR levels in control cells (Ctrl siRNA), lowering HuR, but not lowering AUF1, increased HOTAIR steady-state abundance by more than threefold ( Fig. 2e ). Treatment with Actinomycin D to inhibit transcription revealed that the half-life of HOTAIR , as measured by RT-qPCR-based quantification ( Fig. 2f ), increased from 1.3 h in Ctrl siRNA cells to >3 h in HuR siRNA cells, whereas GAPDH mRNA half-life was unaffected by HuR levels, indicating that HuR selectively lowered HOTAIR stability. In keeping with this notion, HuR overexpression lowered HOTAIR levels ( Fig. 2g ). As shown earlier for lincRNA-p21, human HOTAIR was predicted to associate with several miRNAs, including let7i ( Supplementary Fig. S4a ). These interactions appeared to be functional, as mouse embryonic fibroblasts deficient in Ago2 displayed higher Hotair levels ( Supplementary Fig. S4b ). In HeLa cells, RIP analysis of Ago2 showed extensive enrichment in HOTAIR , while transfection of biotinylated precursor (pre)-let7i followed by pulldown analysis of bound endogenous target RNAs using streptavidin beads and RT-qPCR analysis [14] revealed a strong enrichment in HOTAIR ( Supplementary Fig. S4c ). These interactions affected HOTAIR steady-state levels ( Supplementary Fig. S4d ) and half-life, which increased after silencing Ago2 and declined after overexpressing pre-let7i ( Supplementary Fig. S4e ). RIP analysis revealed that silencing HuR lowered Ago2- HOTAIR complexes ( Supplementary Fig. S4f ). In the presence of an antagomir that inhibits endogenous let7i (AS-let7i), HOTAIR levels increased despite HuR overexpression ( Supplementary Fig. S4g ), whereas overexpression of let7i reversed HOTAIR upregulation by HuR silencing ( Supplementary Fig. S4h ). Collectively, these data indicate that HuR and let7i/Ago2 jointly reduce HOTAIR stability. HOTAIR binds E3 ubiquitin ligases and interaction substrates Both the cytoplasmic and nuclear HOTAIR pools were affected by HuR, as determined by fractionating cells ( Fig. 3a ). Fluorescence in situ hybridization (FISH) analysis confirmed that HOTAIR was found in both the cytoplasm and the nucleus and that HOTAIR abundance rose after HuR silencing ( Fig. 3b ). By RIP analysis, we surveyed numerous RBPs that may interact with HOTAIR , including cytoplasmic RBPs involved in mRNA decay and translation, in miRNA metabolism and in protein ubiquitination [15] ( Supplementary Fig. S1b ). The latter group revealed that two E3 ubiquitin ligases with RNA-binding domains, Mex3b (a RING- and KH domain-containing E3 ubiquitin ligase [16] ) and Dzip3 (a RING- and KKKTK domain-containing E3 ubiquitin ligase [17] ) selectively interacted with HOTAIR ( Supplementary Fig. S1b ). Importantly, the abundance of complexes containing HOTAIR and Dzip3, as well as HOTAIR and Mex3b increased when HuR was silenced, as determined by RIP analysis ( Fig. 3c ; Supplementary Fig. S1a ). As E3 ubiquitin ligases specifically associate with select ubiquitination substrate proteins, we searched for reported Mex3b- and Dzip3-interacting proteins [18] , [19] and focused our attention on those containing RNA-binding domains. RIP analysis revealed that Ataxin-1 (implicated in spinocerebellar ataxia), a protein that specifically associated with Dzip3 (ref. 19 ) and Snurportin-1 (a shuttling protein involved in nucleocytoplasmic transport), which specifically associated with Mex3b (ref. 18 ), each interacted with HOTAIR , particularly when HOTAIR was elevated following HuR silencing ( Fig. 3d ). The approach described in Fig. 2c,d , employing limited RNase T1 digestion followed by RIP analysis of the HOTAIR partial segments, was used to map the regions of interaction of Dzip3, Ataxin-1, Mex3b and Snurportin-1 ( Fig. 3e,f ). For Dzip3 and its ubiquitinated substrate, preferential binding was seen for fragments 11 and 12 (nucleotides ~1,028–1,272), as confirmed in vitro ( Supplementary Fig. S2e,f ); within this segment, Ataxin-1 showed greater binding to fragment 11, Dzip3 to fragment 12 ( Fig. 2d ). For Mex3b, preferred binding was seen in the 5′ region (~125–250), while its interaction substrate, Snurportin-1, associated at an adjacent region (~342–471) and a downstream region (~1,142–1,272). 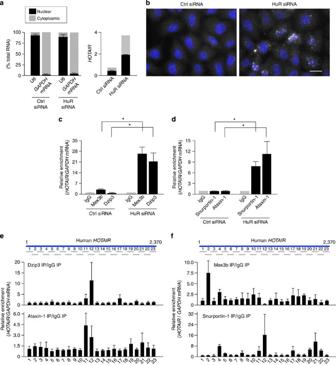Figure 3:E3 ubiquitin ligases and substrates associate withHOTAIR. (a) Forty-eight hours after transfecting HeLa cells with siRNAs, the levels of a nuclear control transcript (U6), a cytoplasmic control transcript (GAPDHmRNA) andHOTAIRwere assessed by RT-qPCR analysis in nuclear and cytoplasmic fractions. (b)HOTAIRFISH analysis (Methods) in HeLa cells processed as described ina. Scale bar, 20 μm. (c,d) Forty-eight hours after siRNA transfection of HeLa cells, the association ofHOTAIRwith endogenous Dzip3 and ectopically expressed Ataxin-1 (c) as well as Mex3b and Snurportin-1 (d) was assessed by RIP analysis using the respective antibodies. (e,f) As explained inFig. 2c and d, the regions of interaction ofHOTAIRwith Dzip3 and Ataxin-1, as well as Mex3b and Snurportin-1, were mapped by partial RNase T1 digestion, followed by RIP analysis of RNA segments enriched in Dzip3 IP (e, top), Ataxin-1 IP (e, bottom), Mex3b IP (f, top) and Snurportin-1 IP (f, bottom) reactions. Ina,candd, the graphs reflect the means and s.d. from three independent experiments; ineandfthe graphs are representative from three independent experiments and show the means and s.d. *P<0.05 using Student’st-test. Figure 3: E3 ubiquitin ligases and substrates associate with HOTAIR . ( a ) Forty-eight hours after transfecting HeLa cells with siRNAs, the levels of a nuclear control transcript ( U6 ), a cytoplasmic control transcript ( GAPDH mRNA) and HOTAIR were assessed by RT-qPCR analysis in nuclear and cytoplasmic fractions. ( b ) HOTAIR FISH analysis (Methods) in HeLa cells processed as described in a . Scale bar, 20 μm. ( c , d ) Forty-eight hours after siRNA transfection of HeLa cells, the association of HOTAIR with endogenous Dzip3 and ectopically expressed Ataxin-1 ( c ) as well as Mex3b and Snurportin-1 ( d ) was assessed by RIP analysis using the respective antibodies. ( e , f ) As explained in Fig. 2 c and d, the regions of interaction of HOTAIR with Dzip3 and Ataxin-1, as well as Mex3b and Snurportin-1, were mapped by partial RNase T1 digestion, followed by RIP analysis of RNA segments enriched in Dzip3 IP ( e , top), Ataxin-1 IP ( e , bottom), Mex3b IP ( f , top) and Snurportin-1 IP ( f , bottom) reactions. In a , c and d , the graphs reflect the means and s.d. from three independent experiments; in e and f the graphs are representative from three independent experiments and show the means and s.d. * P <0.05 using Student’s t -test. Full size image HOTAIR facilitates substrate ubiquitination and degradation Supporting a role for the ubiquitin/proteasome pathway in controlling expression of Ataxin-1 and Snurportin-1, the lowering of Ataxin-1 and Snurportin-1 levels when HuR was silenced (a repression that was linked to the presence of HOTAIR ) was rescued by treatment with the proteasome inhibitor MG132 ( Fig. 4a ). MG132 did not substantially affect Ataxin-1 levels (suggesting slow Ataxin-1 turnover in basal conditions), but it did elevate Snurportin-1 levels ( Fig. 4a ), indicating that the actions of HuR/ HOTAIR to reduce Ataxin-1 and Snurportin-1 required an active proteasome. Interestingly, the interaction of Dzip3 and Ataxin-1, as well as the interaction of Mex3b and Snurportin-1, as assessed by co-IP followed by western blot (WB) analysis, was facilitated by HOTAIR overexpression ( Fig. 4b–d ); furthermore, the levels of Ataxin-1 and Snurportin-1 decreased after HOTAIR overexpression. On the basis of the discovery of these interactions, we hypothesized that HOTAIR might have a new function in protein ubiquitination and protein degradation. 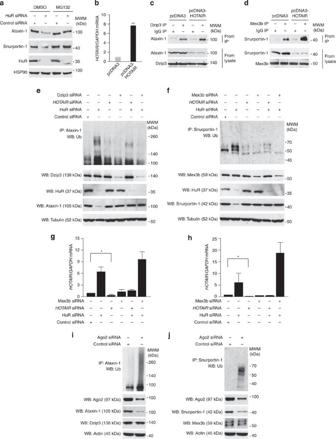Figure 4:HOTAIRpromotes the ubiquitination and degradation of Ataxin-1 and Snurportin-1. (a) HeLa cells were transfected with either Ctrl siRNA or HuR siRNA and 48 h later they were treated with MG132 (20 μM) for 4 h, whereupon the levels of Ataxin-1, Snurportin-1, HuR and loading control HSP90 were assessed by WB analysis. (b–d) Forty-eight hours after overexpressingHOTAIRin HeLa cells (b), the interaction of exogenous Ataxin-1 and endogenous Dzip3 (c), as well as endogenous Snurportin-1 and Mex3b (d), was assessed by IP+WB analysis (‘From IP’); total protein levels in whole-cell lysates were also measured (‘From lysate’). (e,f) Forty-eight hours after transfecting HeLa cells with the siRNAs indicated and with a plasmid to express Ataxin-1 (Methods), the abundance of ubiquitinated Ataxin-1 (e, top) and Snurportin-1 (f, top) was assessed by IP using antibodies that recognized Ataxin-1 or Snurportin-1, followed by ubiquitin WB analysis (Ub); the levels of HuR, Dzip3, Mex3b, Ataxin-1, Snurportin-1 and loading control tubulin were assessed by WB analysis (e,f, bottom). MWM, molecular weight markers. (g,h) RT-qPCR analysis of the abundance ofHOTAIRandGAPDHmRNA in cells treated as ineandf. (i,j) Forty-eight hours after silencing Ago2, the levels of HuR, Dzip3, Mex3b and loading control Actin, as well as Ataxin-1 and ubiquitinated Ataxin-1 (i) and Snurportin-1 and ubiquitinated Snurportin-1 (j), were assessed as explained in panelseandf. Inb,gandh, the graphs reflect the means and s.d. from three independent experiments. *P<0.05 using Student’st-test. Figure 4: HOTAIR promotes the ubiquitination and degradation of Ataxin-1 and Snurportin-1. ( a ) HeLa cells were transfected with either Ctrl siRNA or HuR siRNA and 48 h later they were treated with MG132 (20 μM) for 4 h, whereupon the levels of Ataxin-1, Snurportin-1, HuR and loading control HSP90 were assessed by WB analysis. ( b – d ) Forty-eight hours after overexpressing HOTAIR in HeLa cells ( b ), the interaction of exogenous Ataxin-1 and endogenous Dzip3 ( c ), as well as endogenous Snurportin-1 and Mex3b ( d ), was assessed by IP+WB analysis (‘From IP’); total protein levels in whole-cell lysates were also measured (‘From lysate’). ( e , f ) Forty-eight hours after transfecting HeLa cells with the siRNAs indicated and with a plasmid to express Ataxin-1 (Methods), the abundance of ubiquitinated Ataxin-1 ( e , top) and Snurportin-1 ( f , top) was assessed by IP using antibodies that recognized Ataxin-1 or Snurportin-1, followed by ubiquitin WB analysis (Ub); the levels of HuR, Dzip3, Mex3b, Ataxin-1, Snurportin-1 and loading control tubulin were assessed by WB analysis ( e , f , bottom). MWM, molecular weight markers. ( g , h ) RT-qPCR analysis of the abundance of HOTAIR and GAPDH mRNA in cells treated as in e and f . ( i , j ) Forty-eight hours after silencing Ago2, the levels of HuR, Dzip3, Mex3b and loading control Actin, as well as Ataxin-1 and ubiquitinated Ataxin-1 ( i ) and Snurportin-1 and ubiquitinated Snurportin-1 ( j ), were assessed as explained in panels e and f . In b , g and h , the graphs reflect the means and s.d. from three independent experiments. * P <0.05 using Student’s t -test. Full size image To test this hypothesis, we first examined if HOTAIR affects ubiquitination of associated Ataxin-1, and Snurportin-1. IP of Ataxin-1 or Snurportin-1 followed by ubiquitin WB analysis revealed that silencing HuR increased the pool of ubiquitinated Ataxin-1 and Snurportin-1, identified as high-molecular-weight WB signals (forming discrete or diffuse bands; Fig. 4e,f ; Supplementary Fig. S3a ). Importantly, co-silencing HOTAIR (to 30–40% of the levels in control cells, Fig. 4g,h ) suppressed the effect of HuR silencing in promoting Ataxin-1 and Snurportin-1 ubiquitination ( Fig. 4e,f ); silencing endogenous HOTAIR alone did not affect the ubiquitination of Ataxin-1 or Snurportin-1 likely because basal HOTAIR levels are relatively low and hence unable to modulate ubiquitination in a robust manner. Likewise, Ataxin-1 and Snurportin-1 ubiquitination was inhibited after silencing Dzip3 and Mex3b, respectively ( Fig. 4e,f ; Supplementary Fig. S3c ), even in the presence of elevated HOTAIR levels. The changes in Ataxin-1 or Snurportin-1 did not arise from changes in the encoding mRNAs, as ATXN1 mRNA and SNUPN mRNA levels did not change in the different transfection groups ( Supplementary Figs S3b and S4i,j ). Moreover, silencing Ago2 in HeLa cells, an intervention that elevates HOTAIR ( Supplementary Fig. S4d,e ) increased the ubiquitination of Ataxin-1 and Snurportin-1 and reduced the steady-state levels of these proteins ( Fig. 4i,j ; Supplementary Fig. S3d ), linking Ago2 to the ubiquitination and lower abundance of these two HOTAIR -associated substrates. Together, these data suggest that HuR affects Ataxin-1 and Snurportin-1 ubiquitination in a HOTAIR -dependent manner, and requires E3 ligases Dzip3 and Mex3b, respectively. Second, we tested if ubiquitination of Ataxin-1 and Snurportin-1 in vitro was also dependent on HOTAIR and the corresponding E3 ubiquitin ligases. Using an in vitro ubiquitination system that contained an E1 activating enzyme, an E2 ubiquitin conjugating (Ubc) enzyme (UbcH10 for Ataxin-1 (ref. 20 ), UbcH6 for Snurportin-1; Supplementary Fig. S5a ), and ubiquitin, we performed in vitro ubiquitination in the presence of E3 ligases (Mex3b (recombinant purified) or Dzip3 (immunoprecipitated after expressing Dzip3-FLAG in HeLa cells)), and target RBPs (Ataxin1-1 or Snurportin-1), in the presence or absence of in vitro -synthesized HOTAIR . As shown, HOTAIR increased the ubiquitination of Ataxin-1 by Dzip3 ( Fig. 5a ) and the ubiquitination of Snurportin-1 by Mex3b ( Fig. 5b ); control transcript GAPDH did not promote ubiquitination. The background ubiquitination seen in the reaction samples that did not receive Dzip3 may be due to the fact that E2 enzymes such as UbCH6 can ubiquitinate a substrate with low efficiency in vitro [20] . A systematic analysis of the full complement of E2 ubiquitin-conjugating enzymes and their catalytically inactive variants will be needed to identify the subset of E2 enzymes involved in Ataxin-1 and Snurportin-1 ubiquitination. 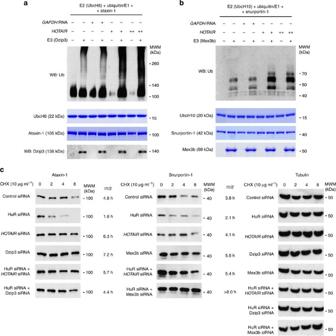Figure 5:HOTAIRpromotes ubiquitinationin vitroand enhances Ataxin-1 and Snurportin-1 degradation. (a,b) The indicated proteins, E1 (ubiquitin), E2 (UbcH6 or UbcH10) and either Ataxin-1 or Snurportin-1, were used in anin vitroubiquitination reaction which also included Dzip3 obtained via IP from HeLa cell lysates (a) or recombinant Mex3b (b); reactions were also supplied withHOTAIRor (control)GAPDHRNA synthesizedin vitro. The abundance of ubiquitinated Ataxin-1 (a) and Snurportin-1 (b) was assessed by WB analysis. (c) Forty-eight hours after transfecting the siRNAs shown, protein stability (t1/2) of Ataxin-1, Snurportin-1 and loading control Tubulin was assessed by measuring the decline of protein levels after CHX treatment. Figure 5: HOTAIR promotes ubiquitination in vitro and enhances Ataxin-1 and Snurportin-1 degradation. ( a , b ) The indicated proteins, E1 (ubiquitin), E2 (UbcH6 or UbcH10) and either Ataxin-1 or Snurportin-1, were used in an in vitro ubiquitination reaction which also included Dzip3 obtained via IP from HeLa cell lysates ( a ) or recombinant Mex3b ( b ); reactions were also supplied with HOTAIR or (control) GAPDH RNA synthesized in vitro . The abundance of ubiquitinated Ataxin-1 ( a ) and Snurportin-1 ( b ) was assessed by WB analysis. ( c ) Forty-eight hours after transfecting the siRNAs shown, protein stability ( t 1/2 ) of Ataxin-1, Snurportin-1 and loading control Tubulin was assessed by measuring the decline of protein levels after CHX treatment. Full size image We then compared the stability of Ataxin-1 and Snurportin-1 in HeLa cells expressing different levels of HuR, HOTAIR and E3 ligases Dzip3 and Mex3b ( Supplementary Fig. S5b ). Silencing HuR rendered Ataxin-1 and Snurportin-1 highly labile, with half-lives of 1.8 and 2.1 h, respectively, as measured by assessing the reduction in protein signals following treatment with the translation inhibitor cycloheximide (CHX) ( Fig. 5c ); the short half-lives were reversed if HOTAIR or E3 ligases (Dzip3 for Ataxin-1, Mex3b for Snurportin-1) were simultaneously reduced ( Fig. 5c ). Whether or not the enhanced ubiquitination and degradation mediated by HOTAIR required the interaction of the protein via the RNA-binding domains and the presence of ubiquitination domains was studied in detail for the Dzip3–Ataxin-1 pair. As shown in Fig. 6a , a mutant Dzip3 (bearing a point mutation in the RING domain, essential for ubiquitination) expressed in HeLa cells from plasmid pTRUF-hRUL138(C1187S) was unable to ubiquitinate Ataxin-1 (top) or promote its degradation (bottom), as compared with the effect of expressing the wild-type counterpart pTRUF-hRUL138(WT) [17] . In addition, ectopic expression of a mutant Ataxin-1(82Q) that cannot bind RNA [21] indeed did not interact with HOTAIR ( Fig. 6b ). Consistent with this observation, Ataxin-1(82Q) was not destabilized by HuR silencing (with t 1/2 changing only from 4.1 to 3.9 h ( Fig. 6c )), in contrast to wild-type Ataxin-1 (bearing 30 Q residues instead), whose t 1/2 changed from 4.8 to 1.8 h after HuR silencing ( Fig. 5c ). Accordingly, the steady-state levels of Ataxin-1(82Q) did not decline after silencing HuR ( Fig. 6d ). Taken together, these data reveal that HOTAIR serves as an assembly scaffold that facilitates the interaction of E3 ligases (Dzip3 and Mex3b) with ubiquitination targets Ataxin-1 and Snurportin-1, respectively. The interaction sites can be proximal (as for Ataxin-1 and Dzip3, HOTAIR fragments 11 and 12 ( Fig. 2d )) or further apart on the linear transcript (as for Snurportin-1 and Mex3b, HOTAIR fragments 12 and 2, respectively ( Fig. 3e,f )). In this regard, overexpression of Ataxin-1 or Snurportin-1 competed for HuR binding to HOTAIR ( Supplementary Fig. S5c ). Of note, HOTAIR did not appear to affect global protein ubiquitination patterns ( Supplementary Fig. S5d ). Together, these results uncover a previously unknown function for a lncRNA as mediator of the ubiquitination and enhanced proteolysis of select proteins ( Fig. 6e ). 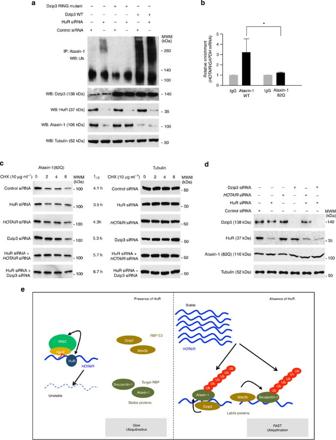Figure 6:HOTAIR-enhanced ubiquitination of Ataxin-1 requires Ataxin-1 binding to the lncRNA and active Dzip3. (a) Forty-eight hours after overexpressing plasmids pTRUF-hRUL138(WT) or pTRUF-hRUL138(C1187S) in HeLa cells, the abundance of ubiquitinated Ataxin-1 (top) was assessed by IP using antibodies that recognized Ataxin-1 followed by ubiquitin WB analysis (Ub); the levels of HuR, Dzip3 (WT and mutant), Ataxin-1 and loading control Tubulin were assessed by WB analysis. MWM, molecular weight markers. (b) Following transfection of HeLa cells with plasmids pCDNA1Amp-ataxin-1(30Q) and pCDNA1Amp-ataxin-1(82Q), RIP analysis was performed to quantify the interaction of WT Ataxin (30Q) and mutant Ataxin (82Q) withHOTAIR; binding was normalized toGAPDHmRNA levels in the IP samples. Data represent the means and s.d. from three independent experiments. (c) Forty-eight hours after transfecting the siRNAs shown and plasmid pCDNA1Amp-ataxin-1(82Q), the stability (t1/2) of Ataxin-1(82Q) and loading control Tubulin was assessed by measuring the decline of protein levels after CHX treatment. (d) By 48 h after transfecting cells as explained inc, the levels of Dzip3, HuR, Ataxin-1(82Q) and loading control Tubulin were assessed by WB analysis. (e) Schematic of the proposed mechanism wherebyHOTAIR, under negative control by HuR, promotes the ubiquitination and degradation of Ataxin-1 and Snurportin-1 by facilitating their assembly with E3 ligases Dzip3 and Mex3b, respectively. Ina,candd, the data are representative from three independent experiments. *P<0.05 using Student’st-test. Figure 6: HOTAIR -enhanced ubiquitination of Ataxin-1 requires Ataxin-1 binding to the lncRNA and active Dzip3. ( a ) Forty-eight hours after overexpressing plasmids pTRUF-hRUL138(WT) or pTRUF-hRUL138(C1187S) in HeLa cells, the abundance of ubiquitinated Ataxin-1 ( top ) was assessed by IP using antibodies that recognized Ataxin-1 followed by ubiquitin WB analysis (Ub); the levels of HuR, Dzip3 (WT and mutant), Ataxin-1 and loading control Tubulin were assessed by WB analysis. MWM, molecular weight markers. ( b ) Following transfection of HeLa cells with plasmids pCDNA1Amp-ataxin-1(30Q) and pCDNA1Amp-ataxin-1(82Q), RIP analysis was performed to quantify the interaction of WT Ataxin (30Q) and mutant Ataxin (82Q) with HOTAIR ; binding was normalized to GAPDH mRNA levels in the IP samples. Data represent the means and s.d. from three independent experiments. ( c ) Forty-eight hours after transfecting the siRNAs shown and plasmid pCDNA1Amp-ataxin-1(82Q), the stability (t 1/2 ) of Ataxin-1(82Q) and loading control Tubulin was assessed by measuring the decline of protein levels after CHX treatment. ( d ) By 48 h after transfecting cells as explained in c , the levels of Dzip3, HuR, Ataxin-1(82Q) and loading control Tubulin were assessed by WB analysis. ( e ) Schematic of the proposed mechanism whereby HOTAIR , under negative control by HuR, promotes the ubiquitination and degradation of Ataxin-1 and Snurportin-1 by facilitating their assembly with E3 ligases Dzip3 and Mex3b, respectively. In a , c and d , the data are representative from three independent experiments. * P <0.05 using Student’s t -test. Full size image HOTAIR levels rise with and contribute to cell senescence As HuR and miRNAs are closely linked to cellular senescence [22] , [23] , we tested if HOTAIR levels were altered during senescence. To study this possibility, we used human IDH4 fibroblasts, which become senescent rapidly after removing dexamethasone (Dex) from the culture medium [22] , and WI-38 human diploid fibroblasts rendered senescent by 10 days after exposure to 10 Gy of ionizing radiation (IR). As reported previously, HuR was lower in senescent cells than in proliferating cells [22] ; interestingly, HOTAIR levels were approximately fourfold higher in senescent cells, whereas Ataxin-1 and Snurportin-1 levels, as well as the levels of Ago2 and TERT, were markedly reduced ( Fig. 7a ). The levels of senescent markers p53, p21 and p16 were elevated ( Fig. 7a ), and cells displayed the characteristic senescence-associated (SA) increase in G1 cell cycle compartment ( Fig. 7b ). FISH analysis confirmed that HOTAIR levels were higher in senescent cells and in cells in which HuR was silenced ( Fig. 7c ). The increased HOTAIR levels were associated with elevated ubiquitination of Ataxin-1 and Snurportin-1 and with lower steady state levels of Ataxin-1 and Snurportin-1 in both senescent models ( Fig. 7d,e ). 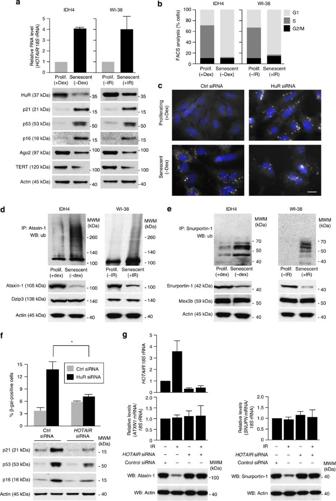Figure 7:HOTAIRpromotes cellular senescence. (a) Five days after removal of Dex from human IDH4 fibroblasts or 10 days after exposure of WI-38 fibroblasts to 10 Gy IR,HOTAIRand18SrRNA levels were measured by RT-qPCR, and the levels of several senescence markers were assessed by WB analysis. ‘Prolif.’, proliferating. (b) Fluorescence-activated cell sorting analysis of proliferating (+Dex, −IR) and senescent cells (−Dex, +IR) to determine the percentage of cells in each cell cycle compartment. The graphs are representative of three independent experiments. (c)HOTAIRFISH analysis in IDH4 cells (+Dex and −Dex) expressing normal (Ctrl siRNA) or reduced (HuR siRNA) levels of HuR. Scale bar, 20 μm. (d,e) The levels of total Ataxin-1 (d) and Snurportin-1 (e) in proliferating and senescent IDH4 and WI-38 cells were detected by WB analysis (IP was included to detect ubiquitinated Ataxin-1 and Snurportin-1, as explained inFig. 4e,f. (f) Cells (%) staining positive for the senescence marker β-galactosidase were counted (top) and senescent marker proteins were assessed by WB analysis (bottom) 48 h after loweringHOTAIRand/or HuR by using siRNAs. (g) Forty-eight hours after loweringHOTAIRin proliferating or senescent WI-38 fibroblasts, the levels ofHOTAIR,ATXN1mRNA andSNUPNmRNA (top), and the levels of Ataxin-1, Snurportin-1 and loading control Actin (bottom) were assessed by RT-qPCR and WB analysis, respectively. Ina,fandg, the graphs reflect the means and s.d. from three independent experiments. *P<0.05 using Student’st-test. Figure 7: HOTAIR promotes cellular senescence. ( a ) Five days after removal of Dex from human IDH4 fibroblasts or 10 days after exposure of WI-38 fibroblasts to 10 Gy IR, HOTAIR and 18S rRNA levels were measured by RT-qPCR, and the levels of several senescence markers were assessed by WB analysis. ‘Prolif.’, proliferating. ( b ) Fluorescence-activated cell sorting analysis of proliferating (+Dex, −IR) and senescent cells (−Dex, +IR) to determine the percentage of cells in each cell cycle compartment. The graphs are representative of three independent experiments. ( c ) HOTAIR FISH analysis in IDH4 cells (+Dex and −Dex) expressing normal (Ctrl siRNA) or reduced (HuR siRNA) levels of HuR. Scale bar, 20 μm. ( d , e ) The levels of total Ataxin-1 ( d ) and Snurportin-1 ( e ) in proliferating and senescent IDH4 and WI-38 cells were detected by WB analysis (IP was included to detect ubiquitinated Ataxin-1 and Snurportin-1, as explained in Fig. 4e,f . ( f ) Cells (%) staining positive for the senescence marker β-galactosidase were counted (top) and senescent marker proteins were assessed by WB analysis (bottom) 48 h after lowering HOTAIR and/or HuR by using siRNAs. ( g ) Forty-eight hours after lowering HOTAIR in proliferating or senescent WI-38 fibroblasts, the levels of HOTAIR , ATXN1 mRNA and SNUPN mRNA (top), and the levels of Ataxin-1, Snurportin-1 and loading control Actin (bottom) were assessed by RT-qPCR and WB analysis, respectively. In a , f and g , the graphs reflect the means and s.d. from three independent experiments. * P <0.05 using Student’s t -test. Full size image That the increased HOTAIR was important for the implementation of senescence was evidenced by experiments in which silencing HOTAIR in IDH4 cells ( Fig. 7f ) reversed the senescent phenotype, with a lower proportion of cells displaying the hallmark SA-β-galactosidase activity along with reduced levels of senescence markers ( Fig. 7f ). Importantly, the reduction in levels of Ataxin-1 and Snurportin-1 in senescent (IR) WI-38 cells was reversed if HOTAIR was silenced ( Fig. 7g ). The lower levels of Ataxin-1 and Snurportin-1 correlated with enhanced ubiquitination of Ataxin-1 and Snurportin-1 ( Fig. 7d,e ); ATXN1 mRNA or SNUPN mRNA levels were unchanged in +Dex compared with −Dex cells ( Supplementary Fig. S6a,b ). In keeping with the lower levels of Ataxin-1 and Snurportin-1 in senescent (−Dex) cells, protein stability was markedly reduced in this group, but the instability was reversed when HOTAIR or the E3 ligases (Mex3b or Dzip3) were silenced ( Fig. 8a,b ). The stability of Ataxin-1 and Snurportin-1 in proliferating (+Dex) cells was also rescued if HuR was silenced, which elevated HOTAIR ( Supplementary Fig. S6c,d ), and was restored if cells were subjected to simultaneous silencing of Dzip3 or Mex3b, respectively ( Fig. 8a,b ). Together, these findings provide a cellular context in which HOTAIR controls gene expression to modulate the protein expression program of senescent cells. 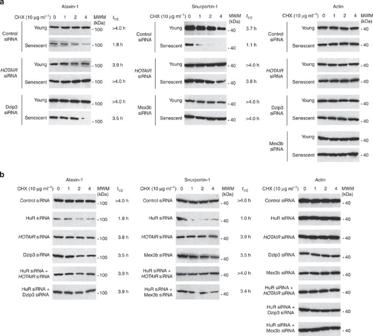Figure 8:HOTAIRaccelerates Ataxin-1 and Snurportin-1 decay in aHOTAIR-, E3 ligase- and senescence-dependent manner. Five days (a) or 48 h (b) after transfecting the siRNAs shown, the stabilities of Ataxin-1 and Snurportin-1 were assessed as explained inFig. 5c; Actin was assessed as loading control. Figure 8: HOTAIR accelerates Ataxin-1 and Snurportin-1 decay in a HOTAIR -, E3 ligase- and senescence-dependent manner. Five days ( a ) or 48 h ( b ) after transfecting the siRNAs shown, the stabilities of Ataxin-1 and Snurportin-1 were assessed as explained in Fig. 5c ; Actin was assessed as loading control. Full size image From these results, a new function emerges for HOTAIR as a possible scaffold transcript that enhances E3-mediated ubiquitination of substrate proteins ( Fig. 6e ). Like other lncRNAs (for example, XIST , ANRIL ), HOTAIR assists in assembling chromatin modification complexes (for example, by recruiting PRC1/2 and LSD-CoREST to repress HOX locus genes) [13] , [24] . The enhanced ubiquitination of Ataxin-1 may be linked to the cytoplasmic presence of HOTAIR , as Dzip3 is localized in the cytoplasm; however, Mex3b and Snurportin-1 are both nuclear and cytoplasmic, suggesting that HOTAIR -facilitated ubiquitination could occur in both compartments. HOTAIR could also participate in other cellular processes via Mex3b, which associates with the signalling protein SMAD4 and with the homoeostasis checkpoint protein NUDT3 (refs 19 , 25 ). The findings that HuR showed preferential binding to a HOTAIR segment spanning nucleotides 1,142–1,272 (fragment 12, Fig. 2d , Supplementary Fig. S2 ) and that this segment was also a strong region of interaction with Dzip3, Ataxin-1 and Snurportin-1 ( Fig. 3e,f ; Supplementary Fig. S2 ), suggests a possible feedback regulatory loop for the levels of the two substrate proteins. According to this model, when Ataxin-1 or Snurportin-1 levels are low, HuR would bind preferentially to HOTAIR , reducing its stability and inhibiting the processes of ubiquitination and proteolysis of Ataxin-1 and Snurportin-1. Conversely, when the levels of the substrate proteins rise, the binding of Ataxin-1, Snurportin-1 or Dzip3 to HOTAIR likely prevents the interaction of HuR with fragment 12, rendering HOTAIR stable and thus facilitating the ubiquitination and degradation of Ataxin-1 and Snurportin-1, as suggested by the finding that Ataxin-1 and Snurportin-1 can displace HuR from HOTAIR ( Supplementary Fig. S5c ). Full experimental support for this putative negative feedback loop awaits further study. In addition, the apparently distal binding of Mex3b, near the 5′ end ( Fig. 3f ), may be understood better after the three-dimensional structure assumed by HOTAIR is elucidated. In the context of cellular senescence, elevated HOTAIR was necessary for eliciting the senescent phenotype ( Fig. 7 ); accordingly, Ataxin-1 and Snurportin-1 were less abundant and less stable in senescent cells ( Fig. 8 ), although the contribution of these proteins (and perhaps other HOTAIR -regulated proteins) in senescence is presently unknown. Senescence is one of the physiologic processes that robustly and permanently lower HuR levels in the cell [22] . However, other cellular processes such as stress responses can transiently lower HuR levels (for example, through cleavage or degradation of HuR [26] , [27] ) or HuR binding to target mRNAs (for example, through phosphorylation of HuR [28] , [29] ). Thus, besides the long-term effect of reduced HuR on HOTAIR -driven ubiquitination and proteolysis seen during senescence, a transient decline in HuR levels or binding to RNA could also temporarily increase a HOTAIR -controlled ubiquitin proteasome pathway in response to cell damage. Our findings add to a growing body of evidence that HuR controls gene expression via a complex network of mediators that includes ncRNAs and other RBPs. In addition to its well-established influence on the stability and translation of mRNAs with which HuR associates directly, HuR can influence protein expression patterns indirectly by facilitating or competing with miRNA function [30] and by controlling the levels of lncRNAs, which in turn elicit other post-transcriptional and post-translational roles. In this regard, HuR was recently shown to downregulate lincRNA-p21, thereby permitting the translation of mRNAs translationally repressed by lincRNA-p21 (ref. 9 ), while our present results show that HuR downregulated HOTAIR , an assembly platform for E3 ubiquitin ligases bearing RNA-binding motifs, Dzip3 and Mex3b, and thus reduced their ability to interact with substrates Ataxin-1 and Snurportin-1. We expect that the rich, multi-levelled post-transcriptional regulation mediated by HuR will also be carried out by other RBPs. In conclusion, together with its scaffold function to assemble transcription regulators, HOTAIR can also serve as a platform to control protein levels via the ubiquitin–proteasome pathway. By acting on multiple levels of gene regulation, HOTAIR and likely other long and short ncRNAs, can robustly influence gene expression programs in physiologic and pathologic states [31] . Anisotropy analysis Untagged recombinant HuR was generated in Escherichia coli ER2566 cells and purified using the IMPACT-CN (Intein Mediated Purification with an Affinity Chitin-binding Tag) system (New England Biolabs) according to manufacturer’s protocol [12] . HuR binding to 3′-fluorescein (Fl)-tagged let7b or let7i (Integrated DNA Technologies) was evaluated by changes in the fluorescence anisotropy of the tagged let7 substrates as a function of protein concentration [12] . Briefly, limiting concentrations of Fl-let7 substrates (0.2 nM) were incubated with varying concentrations of purified HuR in 10 mM Tris-HCl (pH 8.0) containing 50 mM KCl, 2 mM DTT, 0.5 mM EDTA and 0.1 μg μl −1 acetylated bovine serum albumin. Heparin (1 μg μl −1 ) was added to suppress non-specific binding events. Reactions were incubated at room temperature for 30 min before measuring fluorescence anisotropy using a Beacon 2000 Fluorescence Polarization System (Panvera) equipped with fluorescein excitation (490 nm) and emission (535 nm) filters. RNP complex affinity was resolved by nonlinear regression of total measured anisotropy ( A t ) as a function of HuR concentration ([P]) using equation (1) where A R and A PR are the intrinsic anisotropy of the free Fl-let7 and HuR-Fl-let7 complex, respectively, and K is the apparent equilibrium association constant ( K =1/ K d ): The appropriateness of the single-site binding model was evaluated by the coefficient of determination ( R 2 ) from individual experiments and analysis of residual plot non-randomness to detect any bias for data subsets (PRISM v3.03). Analyses of data sets using quadratic binding models incorporating ligand depletion (derived by Wilson [32] ) did not significantly alter resolved HuR-let7 affinity constants. Cell culture and transfection Human HeLa cells (ATCC), human fibroblasts IDH4 (a gift from Dr J.W. Shay, UT Southwestern) and WI-38 (Coriell Cell Repositories), and mouse embryonic fibroblasts (a gift from R. de Cabo, NIA,NIH) were cultured in DMEM (Invitrogen) supplemented with 10% (v/v) fetal bovine serum and antibiotics. For RNA stability assays, HeLa cells were treated with actinomycin D (2.5 μg μl −1 ), followed by RT-qPCR analysis to determine their half-life ( t 1/2 ), the time needed for each transcript to reach 50% of their original abundance. For protein stability assays, cells were treated with CHX (10 μg μl −1 ) for the indicated times and WB analysis followed by densitometry quantification of protein signals was used to measure their half-life ( t 1/2 ), the time necessary for each protein to reach 50% of its original abundance. Cells were transfected (Lipofectamine 2000, Invitrogen) with siRNAs (20 mM) directed to HOTAIR (GAACGGGAGUACAGAGAGAdTdT), HuR (CGUAAGUUAUUUCCUUUAAdTdT), Ago2, Dzip3 and Mex3b (Santa Cruz), with Pre- and anti-let7i (Ambion, 10 nM), or with plasmids. Plasmids that expressed FL and partial HOTAIR transcripts were described previously [13] . Plasmid pCDNA1Amp-ataxin-1[30Q] (a kind gift from H.T. Orr [33] ) was used to overexpress Ataxin-1. Dzip3 was overexpressed from plasmid pTR-UF-hRUL138-FLAG in mammalian cells or from pET-30a-hRUL 832-1176 in E. coli [17] . MBP-HuR was described previously [34] . pHis-GFP-SNP was kindly provided by AG Matera. Transfected cells were generally analysed 48 h later. IDH4 cells were cultured in the presence of 1 mM Dex to preserve the transcription of the SV40 large-T antigen, which suppresses senescence and promotes proliferation. To induce senescence, Dex was removed from the IDH4 culture media, and the regular serum was replaced with charcoal-stripped serum; cells were assessed for senescence 5 days later [22] . For assessment of SA-β-galactosidase activity, cells were seeded in 30-mm diameter dishes, cultured in medium without Dex for 5 days, fixed with a 3% formaldehyde solution, washed and incubated with SA-β-gal staining solution (1 mg ml −1 X-Gal, 40 mM citric acid–sodium phosphate buffer (pH 6.0), 5 mM ferrocyanide, 5 mM ferricyanide, 150 mM NaCl and 2 mM MgCl 2 ) to visualize SA-β-gal activity. WI-38 cells were rendered senescent by exposure to 10 Gy ionizing radiation followed by standard culture for 10 days [35] . Standard fluorescence-activated cell sorting analysis was performed to determine the percentages of G1, S and G2/M cells. Western blot and northern blot analysis Whole-cell lysates, prepared in radioimmunoprecipitation assay (RIPA) buffer, were separated by SDS–polyacrylamide gel electrophoresis, and transferred onto Nitrocellulose membranes (Invitrogen iBlot Stack). Primary antibodies recognizing α-Tubulin, Actin, Ubiquitin, HSP90, HuR, Snurportin-1, Dzip3, Mex3b, p16, p21, p53, TERT and Ataxin-1 were from Santa Cruz Biotechnology (used at 1:1,000 dilution). Antibodies recognizing Ago2, AUF1 and Flag were from Abcam, Millipore and Sigma, respectively (used at 1:1,000 dilution). HRP-conjugated secondary antibodies were from GE Healthcare (used at 1:5,000 dilution). For northern blot analysis, total RNA was prepared by miRNeasy kits (Qiagen) and separated using precast TBE-Urea gel (Invitrogen). Gels were transferred to Nylon membranes (iBlot, Invitrogen) and the membranes were crosslinked using ultraviolet light. DNA oligonucleotides complementary to let-7 or U6 were end-labelled with radioactive ATP and used for probing the nylon membranes [36] . Images were acquired with Typhoon Scanner (GE Healthcare). Larger fields of blots are shown in Supplementary Fig. S7 . RNP analysis For IP of endogenous RNP complexes (RIP analysis) from whole-cell extracts [28] , [36] , cells were lysed in 20 mM Tris-HCl at pH 7.5, 100 mM KCl, 5 mM MgCl 2 and 0.5% NP-40 (and 10 mM N -Ethylmaleimide for ubiquitination assay) for 10 min on ice and centrifuged at 10,000 g for 15 min at 4 °C. The supernatants were incubated with protein A-Sepharose beads coated with antibodies that recognized HuR, Dzip3, Mex3b, Snurportin-1, Ataxin-1 (Santa Cruz Biotechnology), Ago2 (Abcam) or AUF1 (Millipore), or with control IgG (Santa Cruz Biotechnology) for 1 h at 4 °C. After the beads were washed with NT2 buffer (50 mM Tris-HCl at pH 7.5, 150 mM NaCl, 1 mM MgCl 2 and 0.05% NP-40), the complexes were incubated with 20 units of RNase-free DNase I (15 min at 37 °C) and further incubated with 0.1% SDS/0.5 mg ml −1 Proteinase K (15 min at 55 °C) to remove DNA and proteins, respectively. The RNA isolated from the IP materials was further assessed by RT-qPCR analysis using the primers listed ( Supplementary Table S1 ). Normalization of RIP results was carried out by quantifying in parallel the relative levels of U6 snRNA [37] (for RIP analysis of small RNAs) and GAPDH mRNA (for RIP analysis of longer RNA) in each IP sample. These abundant RNAs are non-specific contaminants present in the IP components (microfuge tube, beads, etc.). For mapping experiments, lysates were first digested with RNase T1 (1 units μl −1 , 5 min), whereupon RIP analysis was performed using antibodies that recognized each of the five proteins (HuR, Dzip3, Ataxin-1, Mex3b and Snurportin-1). After washes and isolation of the bound RNA, the segments of HOTAIR bound by each RBP, and hence protected from RNase T1 digestion and immunoprecipitated, were identified by RT-qPCR analysis using primer pairs that scanned the HOTAIR transcript at ~150 nucleotide long, overlapping intervals ( Supplementary Table S1 ). Biotinylated HOTAIR was synthesized using a HOTAIR -expressing plasmid [13] , whereas a biotinylated GAPDH 3′UTR fragment was prepared using as template a T7 promoter-bearing PCR product that contained the GAPDH 3′UTR ( Supplementary Table S1 ). Subcellular fractionation For preparing cytosolic and nuclear fractions, cells were lysed with a buffer containing 10 mM Tris–HCl, pH 7.4, 100 mM, NaCl, 2.5 mM MgCl 2 and 40 μg ml −1 digitonin for 10 min, and the resulting lysates were centrifuged with 2,060 g for 10 min at 4 °C. The supernatant was used for the cytosolic fraction. The pellets were washed, incubated with RIPA buffer at 4 °C for 10 min and the nuclear fraction collected after centrifugation at 4 °C for 10 min at 21,000 g . RT-qPCR analysis Trizol (Invitrogen) was used to extract total RNA and acidic phenol (Ambion) was used to extract RNA for RIP analysis [28] . RT was performed using random hexamers and reverse transcriptase (SSII, Invitrogen) and real-time, quantitative (q)PCR using gene-specific primers ( Supplementary Table S1 and ref. 9 ), and SYBR green master mix (Kapa Biosystems), using an Applied Biosystems 7300 instrument. For miRNA quantitation, RNA extracted from Ago2 and IgG IPs was polyadenylated (System Biosciences, QuantiMiR kit) and hybridized with oligo-dT adaptors. After RT, cDNAs were quantitated by qPCR with miRNA-specific primers or with primers to detect the control transcript U6 , along with a universal primer. FISH analysis Cells were grown in 2-well chambered coverglass (Lab-Tek), briefly washed with PBS, fixed with 4% paraformaldehyde at room temperature for 10 min, washed with PBS and permeabilized in 70% ethanol for >1 h (or stored up to 1 week) at 4 °C; stored cells were briefly rehydrated with Wash Buffer (2 × SSC, 10% formamide) before FISH. The Stellaris FISH Probes to HOTAIR (Biosearch Technologies) were resuspended in hybridization buffer (2 × SSC, 10% formamide, 10% dextran sulphate) to a final concentration of 250 nM per probe set. Hybridization was carried out in a humidified chamber at 37 °C; 16 h later, cells were washed twice (37 °C, 30 min each) with Wash Buffer. The second wash contained 4′,6-Diamidino-2-Phenylindole, Dihydrochloride (DAPI) for nuclear staining (5 ng ml −1 ). The cells were then briefly washed with 2 × SSC, equilibrated with Antifade Buffer (2 × SSC, 0.4% glucose, 10 mM Tris-HCl, pH 8.0) and mounted in freshly prepared Antifade buffer+glucose oxidase+catalase (Sigma) and imaged using a Nikon Eclipse-Ti microscope. In vitro ubiquitination assay The in vitro ubiquitination assay was performed with a kit from Boston Biochemistry. Briefly, E1 (50 nM), E2 UbcHs (50 nM, H6 or H10), E3 enzymes (Dzip3 obtained by IP, and recombinant Mex3b, 100 nM) were incubated with recombinant ubiquitin (200 μM) and substrates (1 μg) at 37 °C for 30 min in reaction buffer containing 50 mM Tris-Cl, pH 7.5, 2.5 mM MgCl 2 , 2 mM DTT and 2 mM ATP [38] . Recombinant E1, E2 and ubiquitin were purchased from Boston Biochem and recombinant Ataxin-1, SNP and Mex3b from Abnova. Additional siRNAs used IDT oligomers (siRNA #2 in each case) rArGrCrGrArArCrCrArCrGrCrArGrArGrArArArUrGrCrAGG (sense) and rCrCrUrGrCrArUrUrUrCrUrCrUrGrCrGrUrGrGrUrUrCrGrCrUrUrU (antisense) were directed to HOTAIR ; rGrArArGrArArGrArGrCrCrUrUrGrUrGrUrGrArUrCrUrGTC (sense) and rGrArCrArGrArUrCrArCrArCrArArGrGrCrUrCrUrUrCrUrUrCrUrU (antisense) were directed to Dzip3, rCrCrArGrGrArUrArCrUrGrCrArGrCrUrUrUrArUrUrArAAG (sense) and rCrUrUrUrArArUrArArArGrCrUrGrCrArGrUrArUrCrCrUrGrGrUrU (antisense) were directed to Mex3b, and rGrArArCrUrArArGrGrArGrCrArGrUrGrGrCrArGrArArGGT (sense) and rArCrCrUrUrCrUrGrCrCrArCrUrGrCrUrCrCrUrUrArGrUrUrCrArG (antisense) were directed at Ago2. UCUUAAGUUUCGUAAGUUAdTdT was directed to HuR. CLIP analysis CLIP analysis was performed by using a shorter (partial) digestion with RNase T1 (ref. 39 ). Briefly, after crosslinking, total HeLa cell lysates were digested with RNase T1 (1 units μl −1 , 5 min) and IP analysis was performed using anti-HuR antibody. After washes and isolation of the bound RNA, the segments of HOTAIR bound by HuR and protected from RNase T1 digestion were subjected to IP and identified by RT-qPCR analysis using primer pairs that scanned the HOTAIR transcript at ~150 nucleotide long, overlapping intervals ( Supplementary Table S1 ). Mapping using CLIP was not possible for HOTAIR -associated RBPs, primarily because of the low abundance of HOTAIR in HeLa cells and in fibroblasts. Only after scaling up substantially the amount of antibody (from 2 to 10 μg per lysate 1mg) and crosslinked lysate (from 3 to 15 mg) were we able to detect a slight crosslink for HuR ( Supplementary Fig. S4b ), but with a great deal of background (not shown). CLIP analysis for the other recombinant proteins and HOTAIR did not detect signals above the high backgrounds seen with these proteins. How to cite this article: Yoon, J.-H. et al. Scaffold function of long non-coding RNA HOTAIR in protein ubiquitination. Nat. Commun. 4:2939 doi: 10.1038/ncomms3939 (2013).